Quadruple perovskite ruthenate as a highly efficient catalyst for acidic water oxidation Development of highly active and durable oxygen-evolving catalysts in acid media is a major challenge to design proton exchange membrane water electrolysis for producing hydrogen. Here, we report a quadruple perovskite oxide CaCu 3 Ru 4 O 12 as a superior catalyst for acidic water oxidation. This complex oxide exhibits an ultrasmall overpotential of 171 mV at 10 mA cm −2 geo , which is much lower than that of the state-of-the-art RuO 2 . Moreover, compared to RuO 2 , CaCu 3 Ru 4 O 12 shows a significant increase in mass activity by more than two orders of magnitude and much better stability. Density functional theory calculations reveal that the quadruple perovskite catalyst has a lower Ru 4d-band center relative to RuO 2 , which effectively optimizes the binding energy of oxygen intermediates and thereby enhances the catalytic activity. Proton exchange membrane water electrolysis (PEMWE) has sparked widely attention as a most promising technology for direct conversion of electrical energy into fuels by electrochemical water splitting [1] , [2] , [3] . Essential to the water electrolyzers is oxygen evolution reaction (OER) taking place at anode, where a complex multistep proton-coupled electron transfer process generates a sluggish kinetics [3] , [4] , [5] . In acid PEMWE, precious-metal oxides of IrO 2 and RuO 2 are currently regarded as the most active OER catalysts [6] . However, high costs and still poor intrinsic activities greatly limit their catalytic efficiencies. Therefore, developing efficient catalysts with less content of precious-metal and higher intrinsic activity is quite appealing for acidic water oxidation. Recently, the synthesis of complex oxides has been reported to be a promising approach for both reducing the precious-metal usage and promoting the intrinsic activity [7] , [8] , [9] , [10] , [11] , [12] , [13] . Various complex oxides with less precious-metal contents, including perovskite [7] , [8] , [9] , [10] and pyrochlore-type [11] , [12] , [13] compounds, were found to exhibit higher intrinsic OER activities relative to the simple binary oxides under acid conditions. For instance, the specific activity reached to about 2.8 mA cm −2 oxide at 1.55 V for perovskite oxide Ba 2 NdIrO 6 , which is about 14 times larger than that of the commercial IrO 2 ( ∼ 0.2 mA cm −2 oxide ) [8] . A more efficient IrO x /SrIrO 3 catalyst with a high specific current density of 10 mA cm −2 oxide at 1.50 V was revealed by strontium leaching from surface layers of SrIrO 3 thin films during electrochemical testing [9] . Similar promotions were also observed in pyrochlore-type Y 2 Ir 2 O 7 and Y 2 Ru 2 O 7-δ catalysts [12] , [13] . Compared to iridium, ruthenium is much lower in price [4] , [6] , [13] . Moreover, ruthenium oxide typically exhibits higher activity than iridium oxide [4] , [6] . Therefore, the ruthenium oxides with complex structures represent promising catalysts for acidic water oxidation. In this work, we report a complex perovskite oxide CaCu 3 Ru 4 O 12 as a highly efficient catalyst for OER in acid. Unexpectedly, this ruthenate catalyst presents an ultralow overpotential of 171 mV at 10 mA cm −2 geo in 0.5 M H 2 SO 4 solution, surpassing the most reported robust OER catalysts in acid up to date. Moreover, it achieves large mass activity of 1942 A g −1 Ru and specific activity of 22.1 mA cm −2 oxide at 1.50 V, which are 170 and 96 times higher than those of the commercial RuO 2 , respectively. The long-term durability tests also reveal that CaCu 3 Ru 4 O 12 shows much better stability than RuO 2 . The excellent OER performance of this ruthenate oxide would make it a promising catalyst in commercial PEMWE. Synthesis and characterization The ruthenate oxide CaCu 3 Ru 4 O 12 belongs to the typical A-site ordered quadruple perovskite compound AA' 3 B 4 O 12 , whose crystal structure can be considered as a 2 × 2 × 2 superstructure of simple cubic perovskite ABO 3 . As shown in Fig. 1a , one Ca 2+ and three Cu 2+ ions occupy A-sites in order, while the Ru 4+ ions form corner-share RuO 6 octahedra at B-sites [14] , [15] . The polycrystalline powders of this compound were synthesized by a conventional solid-state reaction. Scanning electron microscopy (SEM) image displays that the particle sizes are submicron (Supplementary Fig. 1 ). 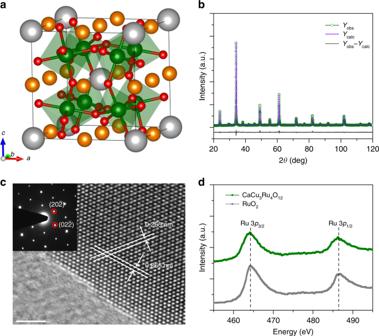Fig. 1 Structural characterization of CaCu3Ru4O12.aCrystal structure of CaCu3Ru4O12. Color code: Ca (gray), Cu (bronze), Ru (green), and O (red).bXRD pattern for CaCu3Ru4O12together with the Rietveld refined results.cHRTEM image and SAED pattern (inset) for CaCu3Ru4O12. The scale bar is 2 nm.dRu 3p XPS spectra Figure 1b shows the powder X-ray diffraction (XRD) of as-prepared sample, where all the diffraction lines are well indexed to the cubic ( Im-3 ) phase without detectable amount of impurities. On the base of Rietveld refinements on diffraction data, the lattice parameter a and Ru–O bond length are determined to be 7.4206(3) and 1.9808(7) Å (Supplementary Table 1 ), respectively, which well agrees with the reported values [14] . The good crystallinity and single-phase structure are further confirmed by high resolution transmission electron microscopy (HRTEM) image together with selected area electron diffraction (SAED) pattern (Fig. 1c ). The observed lattice fringes with inter-plane spacing of 0.265 nm correspond to the \(\left( {02\bar 2} \right)\) or \(\left( {20\bar 2} \right)\) plane of cubic phase CaCu 3 Ru 4 O 12 . X-ray photoelectron spectra (XPS) measurements (Fig. 1d ) reveal that CaCu 3 Ru 4 O 12 exhibits two peaks at 464.2 and 486.3 eV, which are similar to those of RuO 2 and assigned to 3p 3/2 and 3p 1/2 states of Ru 4+ ions [16] , respectively. The energy dispersive X-ray spectrum (EDS, Supplementary Fig. 2 ) demonstrates that the molar ratio of Ca/Cu/Ru is 1:2.98:4.03, which suggests a good stoichiometry of the as-synthesized sample. Fig. 1 Structural characterization of CaCu 3 Ru 4 O 12 . a Crystal structure of CaCu 3 Ru 4 O 12 . Color code: Ca (gray), Cu (bronze), Ru (green), and O (red). b XRD pattern for CaCu 3 Ru 4 O 12 together with the Rietveld refined results. c HRTEM image and SAED pattern (inset) for CaCu 3 Ru 4 O 12 . The scale bar is 2 nm. d Ru 3p XPS spectra Full size image OER performance We evaluated the electrocatalytic OER activity of CaCu 3 Ru 4 O 12 in O 2 -saturated 0.5 M H 2 SO 4 solution using a standard three-electrode system. 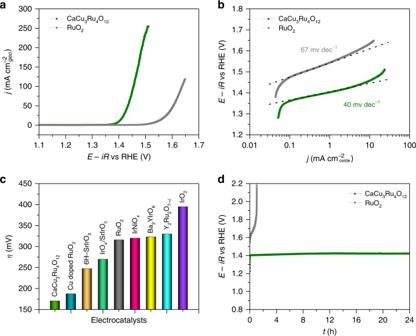Fig. 2 Electrochemical OER performance.aPolarization curves of CaCu3Ru4O12and the commercial RuO2measured in O2-saturated 0.5 M H2SO4solution.bTafel plots of specific OER activity.cComparison of the overpotentials at 10 mA cm−2geofor CaCu3Ru4O12and recent reported OER catalysts in acid media.dChronopotentiometric measurements of CaCu3Ru4O12and the commercial RuO2at 10 mA cm−2geo Figure 2a shows the polarization curve for CaCu 3 Ru 4 O 12 , along with the commercial RuO 2 as a reference. For RuO 2 , a large overpotential ( η ) of 316 mV was required to achieve a current density of 10 mA cm −2 geo , which is in line with those previous reports (Supplementary Table 2 ). Intriguingly, for CaCu 3 Ru 4 O 12 , the current density is remarkably enhanced and the overpotential is much reduced to 171 mV. Moreover, by normalizing the current density to catalyst mass or Ru metal mass, a significant increase in the mass activity is observed (Supplementary Fig. 3 ). For example, the mass activity of CaCu 3 Ru 4 O 12 achieves 1942 A g −1 Ru at 1.50 V, which is 170 times higher than that of RuO 2 (11.4 A g −1 Ru ). As shown by Tafel plots in Fig. 2b , this enhanced performance is further verified to be intrinsic by the specific activity, which is obtained from normalizing the mass activity with Brunauer-Emmett-Teller (BET) surface area (Supplementary Fig. 4 ). Notably, the specific current density of CaCu 3 Ru 4 O 12 at 1.50 V reaches up to the value of 22.1 mA cm −2 oxide , which is 96 times larger than that of RuO 2 (0.23 mA cm −2 oxide ). The similar feature is also found in the specific activities normalized by the electrochemically active surface areas (ECSA), which are derived from the electrochemical double-layer capacitance measurements (Supplementary Fig. 5 , 6 ). Meanwhile, the Tafel plots illustrate that CaCu 3 Ru 4 O 12 presents a smaller Tafel slope of 40 mV dec −1 than RuO 2 of 67 mV dec −1 , suggesting its significantly accelerated OER kinetic. The faster OER kinetic rate is further reflected by the electrochemical impedance spectroscopy (EIS) measurements, where a remarkable decrease of charge transfer resistance (Rct) is revealed for the ruthenate catalyst (Supplementary Fig. 7 ). Fig. 2 Electrochemical OER performance. a Polarization curves of CaCu 3 Ru 4 O 12 and the commercial RuO 2 measured in O 2 -saturated 0.5 M H 2 SO 4 solution. b Tafel plots of specific OER activity. c Comparison of the overpotentials at 10 mA cm −2 geo for CaCu 3 Ru 4 O 12 and recent reported OER catalysts in acid media. d Chronopotentiometric measurements of CaCu 3 Ru 4 O 12 and the commercial RuO 2 at 10 mA cm −2 geo Full size image Our electrochemical tests clearly demonstrate that CaCu 3 Ru 4 O 12 exhibits a superior activity for acidic water oxidation. To the best of our knowledge, this complex oxide has the lowest overpotential at 10 mA cm −2 geo among the excellent OER catalysts in acid electrolytes as reported up to date (Fig. 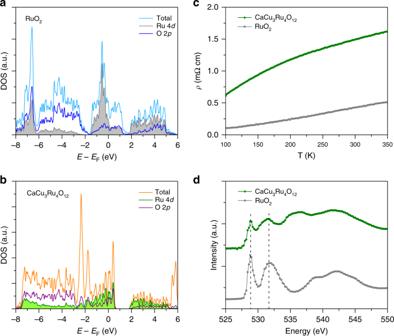Fig. 3 Electronic structure studies.a, bComputed density of states (DOS) ofaRuO2andbCaCu3Ru4O12.cTemperature dependence of resistivity.dOK-edge XAS 2c and Supplementary Table 3 ). Furthermore, its intrinsic activity also outperforms all of them. Particularly, the specific current density of the ruthenate at 1.50 V is even about two-fold higher than that of the recently reported best oxide catalyst IrO x /SrIrO 3 (Supplementary Table 3 ). To access the electrochemical stability of CaCu 3 Ru 4 O 12 , we performed a long-term chronopotentiometry at a constant current density of 10 mA cm −2 geo , together with RuO 2 for comparison. As shown in Fig. 2d , the commercial RuO 2 nearly loses all its activity after 1 h. In constrast, the overpotential for CaCu 3 Ru 4 O 12 just slightly increases from 171 to 192 mV after a 24 h continuous operation. The high stability of this complex oxide is also supported by the XRD, XPS, and HRTEM measurements after the OER test. No visible changes in the positions of XRD diffraction lines and XPS core level peaks (Supplementary Fig. 8 ) are found on the materials before and after the OER testing, while there is a marked decrease in the intensities due to the less catalyst mass used in the measurements after the OER testing. HRTEM image (Supplementary Fig. 9 ) further shows that the lattice fringes for the CaCu 3 Ru 4 O 12 particle after the durability test still extend all the way to the surface, which suggests that the surface structure of CaCu 3 Ru 4 O 12 is maintained during OER. 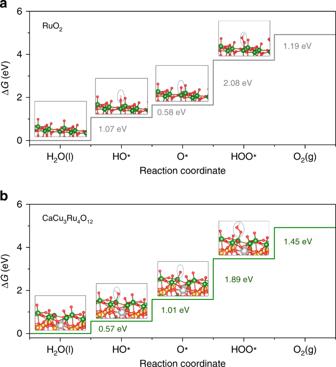Fig. 4 Calculated free energy diagrams.aRuO2.bCaCu3Ru4O12. The optimized structures of HO*, O*, and HOO* adsorptions on the surfaces are shown in the insets In addition, inductively coupled plasma atomic emission spectroscopy (ICP-AES) measurements (Supplementary Table 4 ) reveal that less than 6.7% Ca, 2.9% Cu, and 2.7% Ru ions are found to be dissolved in the electrolyte, indicating just a slight cation leaching during the OER operation. This is also confirmed by TEM-EDS spectrum (Supplementary Fig. 10 ), which shows a small change of Ca/Cu/Ru ratio for ruthenate catalyst after the acidic OER testing. These results suggest that this ruthenate oxygen-evolving catalyst shows good chemical stability in acid, which will be beneficial for the commercial applications. To understand the enhanced OER activity in the complex oxide CaCu 3 Ru 4 O 12 , density functional theory (DFT) calculations were carried out. Figures 3a, b show the computed density of states (DOS) for RuO 2 and CaCu 3 Ru 4 O 12 , respectively. The large DOS from Ru 4d and O 2p bands cross the Fermi level for both the oxides, which indicates that they present an intrinsically metallic behavior. However, compared to RuO 2 , CaCu 3 Ru 4 O 12 exhibits a downshift in the projected DOS for both Ru 4d band and O 2p band relative to the Fermi level. For RuO 2 , the calculated Ru 4d band and O 2p band centers are 0.72 and 0.16 eV, while the values are reduced to −1.37 and −3.42 eV for CaCu 3 Ru 4 O 12 , respectively. To confirm these electronic features, we further conducted the electrical transport measurements. Figure 3c plots the temperature-dependent resistivity for RuO 2 and CaCu 3 Ru 4 O 12 . Upon cooling, their electrical resistivities show a monotonous decrease. This temperature dependence reveals an intrinsic metallic state for both the oxides, agreeing well with the DFT calculations. The metallic conductivity could ensure fast charge transfer between catalyst-electrolyte and catalyst-support electrode interfaces, which is beneficial for the OER process [17] . Moreover, the resistivity of CaCu 3 Ru 4 O 12 is apparently higher than that of RuO 2 within the measured temperature range. For example, CaCu 3 Ru 4 O 12 exhibits a more than threefold increase in the resistivity (1.5 mΩ cm) at room temperature compared to RuO 2 (0.43 mΩ cm). The larger resistivity is supposed to be associated with the Ru 4d and O 2p band centers far away from the Fermi level owing to their downshifts to low energies. Fig. 3 Electronic structure studies. a, b Computed density of states (DOS) of a RuO 2 and b CaCu 3 Ru 4 O 12 . c Temperature dependence of resistivity. d O K -edge XAS Full size image During the OER process, the conventional adsorbate mechanism demonstrates that the electrochemical activity of catalysts is determined by the binding strengths of adsorbed intermediates such as HO*, O*, and HOO* to active sites [18] , [19] , [20] , [21] , [22] . For transition metal oxide OER catalysts, the d-band center of active metal sites is closely related to the binding strength between metal sites and adsorbed oxygen species [22] , [23] , [24] . Usually, a lower d-band center generates a weaker metal-oxygen binding [22] , [23] , [24] . In our case, the refined Ru–O bond length of CaCu 3 Ru 4 O 12 is 1.9808(7) Å, which is longer than the average Ru–O bond length of RuO 2 (~1.97 Å) [25] , [26] . This implies that CaCu 3 Ru 4 O 12 has a weaker Ru–O bonding strength compared to RuO 2 , well associated with that the former has a lower Ru 4d-band center. To further assess the strength of Ru–O bonds in our catalysts, we performed the O K-edge X-ray absorption spectroscopy (XAS). O 1 s spectra in K-edge XAS reflect the transition from O 1 s core level to unoccupied O 2p states hybridized with metal ions [27] , [28] . A higher absorption intensity of O 1 s spectra suggests a stronger hybridization between oxygen and metal ions. As shown in Fig. 3d , two pre-edge peaks are clearly observed at 528.8 and 531.7 eV for our catalysts, which are assigned to the unoccupied orbitals of O 2p hybridized with Ru 4d t 2g and e g orbitals [29] , [30] , respectively. The intensities of pre-edge peaks normalized by the adsorption background at the energy ranges both below the absorption edge and at ∼ 550 eV [27] , [28] , [31] are used to estimate the hybridization of O 2p with Ru 4d orbitals. Obviously, the normalized intensities for CaCu 3 Ru 4 O 12 are much smaller than those for RuO 2 , which implies that the Ru–O bonds in the complex oxide have a less hybridization. This feature further supports that a weaker Ru–O binding strength occurs in CaCu 3 Ru 4 O 12 owing to its lower Ru 4d band center. To elucidate the role of the electronic structures on OER energetics for our Ru-based oxides, theoretical OER overpotentials were further evaluated from DFT calculations. According to the previous studies [18] , [19] , [20] , [21] , [22] , we assumed a four-step OER mechanism, which proceeds through four consecutive proton and electron transfer steps with HO*, O*, and HOO* intermediates. The Gibbs free energies of different intermediates adsorbed by surface Ru atoms for both catalysts were calculated with the standard hydrogen electrode (SHE) method [32] , [33] . Firstly, we focused on RuO 2 (110) and CaCu 3 Ru 4 O 12 (001) surfaces (Supplementary Fig. 11 , 12 ), since they are considered as the relatively more stable facets for rutile and pervoskite oxides [16] , [19] , [20] , respectively. Figure 4a, b illustrates the free energy diagrams calculated on both the surfaces. For RuO 2 , all reaction steps move uphill in free energy at zero potential. Moreover, the free energy difference between Δ G HOO* and Δ G O* is found to be maximum, i.e., Δ G HOO* − Δ G O* = 2.08 eV, indicating that a minimum potential of U = 2.08 V has to be applied to make every step downhill in free energy. This means that the formation of HOO* from O* intermediates is the rate-determining step (RDS), which results in a high OER overpotential of 0.85 V. Our calculations on RuO 2 are in accord with previous reports [16] , [34] , [35] . For CaCu 3 Ru 4 O 12 , the formation of HOO* intermediates is still the RDS. However, Δ G HOO* − Δ G O* is significantly reduced to 1.89 eV, corresponding to a theoretical overpotential of 0.66 V. These calculated results imply that compared to RuO 2 the quadruple perovskite ruthenate exhibits a much reduction in the OER overpotential by 0.19 V. Notably, our calculated OER overpotentials are different from the experimental values possibly because the formers are just obtained from the thermodynamic analyses [10] . However, the magnitude of reduction in the overpotentials is comparable between them (0.19 V vs 0.145 V), which supports that the unique electronic structure associated with the quadruple perovskite crystal structure for CaCu 3 Ru 4 O 12 would be responsible for the observed superior OER activity. Fig. 4 Calculated free energy diagrams. a RuO 2 . b CaCu 3 Ru 4 O 12 . The optimized structures of HO*, O*, and HOO* adsorptions on the surfaces are shown in the insets Full size image Additionally, we also carried out the DFT calculations on other facets for both the catalysts. For RuO 2 , as shown in Supplementary Fig. 13 , 14 , the free energy diagrams for less stable (001) and (100) surfaces illustrate that the theoretical overpotentials are 1.00 and 0.74 V, respectively, which are still larger than that of CaCu 3 Ru 4 O 12 (001) surface. For CaCu 3 Ru 4 O 12 , the calculations on (110) surface (Supplementary Fig. 15 ) reveal that this high-index facet exhibits an inferior OER activity with a theoretical overpotential of 0.85 V. Furthermore, in order to evaluate the role of Ca and Cu cations on the OER activity, we calculated the free energy diagrams on Ca and Cu sites for CaCu 3 Ru 4 O 12 (001) surface, as shown in Supplementary Fig. 16 , 17 . The theoretical overpotentials are estimated to be 0.99 and 0.92 V, respectively, which both are much larger than that on Ru sites (0.66 V). This result strongly supports that Ru cations are the OER active sites for CaCu 3 Ru 4 O 12 . Recent theoretical studies on the OER mechanism for transition metal oxides have demonstrated that the Δ G O* − Δ G HO* difference can effectively describe their OER activities since there is a strong relations between Δ G HO* and Δ G HOO* [19] , [20] , [21] , [22] . Actually, this difference reflects the metal-oxygen binding strength [22] . The optimal catalysts are required to have neither too strong nor too weak binding strengths. Too strong metal-oxygen bond strength would result in a small Δ G O* − Δ G HO* difference and then a large Δ G HOO* − Δ G O* difference. Our DFT calculations reveal CaCu 3 Ru 4 O 12 exhibits a much reduction in Δ G HOO* − Δ G O* difference with comparison to RuO 2 . Moreover, this reduction is accompanied by a large increase in Δ G O* − Δ G HO* from 0.58 to 1.01 eV. In other words, the weaker Ru–O coupling in CaCu 3 Ru 4 O 12 leads to a larger Δ G O* − Δ G HO* and then a smaller Δ G HOO* − Δ G O* , i.e., a smaller overpotential. Therefore, we conclude that the weaker binding strength between oxygen species and Ru sites due to the lower Ru 4d band center gives rise to the higher intrinsic activity of quadruple perovskite CaCu 3 Ru 4 O 12 . In addition, previous studies revealed that the instability for RuO 2 may be attributed to the high Ru dissolution rate due to oxygen vacancies arising from the participation of activated lattice oxygen in OER process [36] . For transition metal oxides, the strong metal-oxygen couplings were reported to easily trigger the lattice oxygen redox during OER [37] . We thus suppose that the weaker Ru–O binding strength in CaCu 3 Ru 4 O 12 may also lower the Ru dissolution rate owing to the less participation of lattice oxygen redox in the OER process, which will improve its stability in acid. In summary, we develop a complex ruthenate CaCu 3 Ru 4 O 12 as an efficient OER catalyst with excellent activity and good durability in acidic media. It only requires an ultralow overpotential of 171 mV to yield a current density of 10 mA cm −2 geo under pH = 0. The mass activity reaches up to 1942 A g −1 Ru at 1.50 V, which is 170 times higher than that of the state-of-the-art RuO 2 . Moreover, this complex oxide exhibits much better stability than RuO 2 . Electronic structure studies and DFT calculations reveal that compared to that of RuO 2 , the adsorption of oxygen intermediates for CaCu 3 Ru 4 O 12 is significantly weakened due to its lower Ru 4d-band center, which facilitates the sluggish kinetics of oxygen-evolving process and enhances the intrinsic activity. This work not only demonstrates that the quadruple perovskite ruthenate holds great potential in the commercial application of PEMWE, but also provides a guidance for exploiting superior oxygen-evolving catalysts from the materials with complex structures. Synthesis and characterizations The polycrystalline powders of quadruple perovskite oxide CaCu 3 Ru 4 O 12 were prepared by a conventional solid-state reaction. Stoichiometric mixtures of 0.2002 g CaCO 3 , 0.4773 g CuO, and 1.0645 g RuO 2 were thoroughly ground and sintered in static and ambient air at 1000 °C for 24 h. Then, the obtained powders were reground and calcined in static and ambient air at 1000 °C for 24 h to produce the sample. All the products were furnace-cooled to room temperature and ground by hand. The powder XRD patterns were collected on a Rigaku TTR-III diffractometer equipped with a Cu Kα radiation source (λ = 1.5418 Å). The SEM images were obtained on the field emission scanning electron microscope (JEOL-2010 SEM) operated at 5 kV. The SEM specimens were prepared by depositing the catalyst powders on conductive carbon adhesive tape. HRTEM images and SAED patterns were acquired using a transmission electron microscope (JEOL, JEM-ARM200F) with a spherical aberration corrector at an acceleration voltage of 200 kV. For TEM specimen preparation, the catalyst powders were firstly dispersed in ethanol by sonication and then dropped onto a carbon-coated molybdenum grid with micropipettes, followed by drying under ambient conditions. XPS were carried out on an ESCALAB 250 X -ray photoelectron spectrometer using an Al Kα X-ray source. For XPS analysis, the binding energies were calibrated by referencing the C 1 s peak to 284.8 eV and no background subtraction was performed. The nitrogen adsorption-desorption isotherms were recorded at 77 K according to the preset pressure procedure using a Micromeritics ASAP 2000 system. Prior to the measurements, the samples were outgassed at 300 °C under vacuum for 10 h. The total surface areas were deduced from the isotherm analysis over the range of the relative pressure from 0.05 to 0.20. ICP-AES was performed on a Perkin-Elmer Optima 3300DV ICP spectrometer. The temperature-dependent resistivities of pelleted samples were measured on a Quantum Design Physical Property Measurement System by using the four-probe method. O K -edge XAS were measured at the beamline BL12B of National Synchrotron Radiation Laboratory (NSRL, Hefei) in the total electron yield mode by collecting the sample drain current under a vacuum better than 10 −7 Pa. The beam from the bending magnet was monochromatized by utilizing a varied line-spacing plane grating and refocused by a toroidal mirror. The spectra from 525 to 550 eV were scanned with an energy resolution of 0.2 eV. To eliminate the effect of different sample concentration and measurement conditions on the intensity of XAS peaks, all the spectra were normalized to the adsorption background at the energy ranges both below the absorption edge and at ∼ 550 eV as described in the literatures [27] , [28] , [31] . The XAS specimens were prepared by placing a small amount of catalyst powders on a conductive carbon tape, which was mounted on an aluminum holder attached to the main chamber manipulator. Electrochemical measurements The electrochemical tests were performed with a three-electrode on the CHI660E electrochemical station. Saturated Hg/Hg 2 SO 4 and platinum wires were used as the reference and the counter electrodes, respectively. The Hg/Hg 2 SO 4 reference electrode was calibrated in H 2 -saturated 0.5 M H 2 SO 4 solution with a Pt wire as working electrode. The measured potentials vs Hg/Hg 2 SO 4 were converted to the values with reference to a reversible hydrogen electrode (RHE). In 0.5 M H 2 SO 4 , E RHE = E Hg/Hg2SO4 + 0.652 V. To prepare the working electrode, the catalysts (18.5 mg), activated carbon (3.7 mg), and Nafion (5 wt%, 100 μL) were dispersed in 5 mL tetrahydrofuran (THF) with sonication for 30 min to generate a homogenous ink. Then 5 μL ink was drop-casted onto a glassy carbon electrode of 3 mm in diameter and dried naturally, yielding a catalyst loading of 0.25 mg cm −2 . Linear sweeping voltammograms were obtained at a scan rate of 5 mV s −1 . The potentials are іR -corrected to compensate for the effect of solution resistance, which were calculated by the following equation: 
    E_iR - corrected = E - iR,
 (1) where i is the current, and R is the uncompensated ohmic electrolyte resistance (~8 Ω) measured via high frequency ac impedance in O 2 -saturated 0.5 M H 2 SO 4 solution. EIS measurements were carried out at different potential values with the frequency ranging from 100 kHz to 100 mHz under an AC voltage of 5 mV. The impedance spectra were presented in the form of Nyquist plot and fitted using ZView software with a representative equivalent electrical circuit. ECSA was determined by measuring the capacitive current associated with double-layer charging from the scan-rate dependence of cyclic voltammetry (CV) [10] , [17] . The potential window of CV was set to be 1.21–1.31 V vs RHE and the scan rates were 10, 20, 40, 60, 80, and 100 mV s −1 . The double-layer capacitance (C dl ) was estimated by plotting the Δj = (j + − j − )/2 at 1.26 V vs RHE against the scan rate. The ECSA was calculated by the following equation: 
    ECSA = ( C_dl/C_s)/M,
 (2) where C s and M represented the specific capacitance and the loading mass for the catalyst, respectively. A C s value of 60 μF cm −2 was used as the common estimate for oxide surfaces [38] , [39] . To conduct the long-term chronopotentiometric measurements, the catalysts were deposited on carbon paper with a mass loading of 0.25 mg cm −2 and followed by a heat-treating in ambient air at 300 °C. To carry out XRD and XPS measurements after the durability test for the catalysts, we followed the approaches frequently reported in recent literatures [7] , [12] , [13] , where the catalysts were loaded onto carbon paper with a high loading of 1 mg cm −2 for the durability test. After washing with ethanol and sonication, the specimens of ~2 mg were collected to use. Computational methods All the density functional theory (DFT) calculations were performed with the Vienna Ab-initio Simulation Package (VASP). The projector augmented wave (PAW) potentials and Perdew-Burke-Ernzerhof (PBE) exchange-correlation functional were adopted. All calculations were conducted using a plane-wave kinetic energy cutoff of 520 eV. The energy convergence criterion was set to be 10 −5 eV, and the force on each ion was converged to less than 0.05 eV/Å. The relevant details, models, and references are given in the Supplementary Methods section.